Insight into the early evolution of the avian sternum from juvenile enantiornithines The sternum is one of the most important and characteristic skeletal elements in living birds, highly adapted for flight and showing a diverse range of morphologies. New exceptional material of young juvenile specimens from the Early Cretaceous Jehol Group in northeastern China reveals the unique sequence of development in the sternum of Enantiornithes, the dominant clade of Cretaceous birds. We recognize six ossifications that together form the sternum, three of which were previously unknown. Here we show that although basal living birds apparently have retained the dinosaurian condition in which the sternum develops from a bilateral pair of ossifications (present in paravian dinosaurs and basal birds), the enantiornithine sternal body primarily develops from two unilateral proximo-distally arranged ossifications. This indicates that although superficially similar, the sternum formed very differently in enantiornithines and ornithuromorphs, suggesting that several ornithothoracine sternal features may represent parallelism. This highlights the importance of ontogenetic studies for understanding homology and the evolution of skeletal features in palaeontology. Unlike the sternal bones in other living animal groups, the massive keeled sternum that characterizes flying birds is one of the most distinctive skeletal features of the group, attesting to its highly specialized purpose [1] . The sternum is the largest bone in the modern avian skeleton; it has many functions, almost of all of which are thought to be related to flight, and thus, it is typically reduced and without a keel (carina) in flightless taxa (for example, living ratites, Cretaceous Hesperornis ) [1] , [2] . This large bone provides attachment surface for the powerful flight muscles, the m. supracoracoideus and m. pectoralis ; the former contributes to lifting the wing during flight and is especially important during take-off, whereas the latter is primarily responsible for the downstroke [1] . These large muscles typically account for 25–35% of the average neornithine body mass [1] , [3] . Although treated as a single bone, the sternum is actually a synstotic element formed by pairs of unilateral and bilateral homologous elements [4] , [5] , [6] , [7] , [8] and may represent one of the most complex elements in the avian skeleton. However, an ossified sternum was completely absent in the most basal bird, Archaeopteryx , despite its presence in several groups of non-avian maniraptoran dinosaurs considered close relatives to birds (Dromaeosauridae, Oviraptorosauria; see Methods; Supplementary Fig. S1 ). Sternal complexity comparable to living birds (for example, caudally extending processes, ventrally projecting carina) only appears in Ornithothoraces, the clade that includes Enantiornithes, the dominant group during the Cretaceous, and Ornithuromorpha, the group that includes living taxa (Neornithes). When present, basal avian taxa (Confuciusornithiformes) possessed simple, plate-like morphologies comparable to the sterna of closely related dinosaurs such as oviraptorosaurs ( Citipati osmolska ) and dromaeosaurids ( Microraptor gui ). With all major clades of Mesozoic birds appearing simultaneously in the Early Cretaceous, intervening stages are poorly known, and the development and evolution of the complex sternum has until now been largely unknown. Ontogenetic information can clarify phylogenetic hypotheses and provide insight into the evolution of a feature [9] , [10] ; unfortunately, specimens that record the early ontogenetic stages of extinct taxa are extremely rare. However, the rich Early Cretaceous Jehol Group lagerstätten has revealed a number of juvenile enantiornithine birds representing a unique wealth of data on the early evolution of Aves. Here we report on several new specimens of exceptionally well-preserved early juvenile enantiornithines that, together with previously described specimens, document the development of the sternum in this clade. These specimens show how the sternum, like in living birds, is a complex bone formed by several elements. Comparison with the morphology of the sternum in non-avian dinosaurs and the development of the sternum in living birds reveals major differences in the development of this element. This may suggest that shared features of the sternum are parallelisms (not developmentally homologous, see Supplementary Information ), highlighting the large amount of homoplasy that characterizes avian evolution as a result of the constraints of powered flight. Systematic palaeontology Aves Ornithothoraces Enantiornithes indet. Referred specimens . STM 34-1 ( Figs 1c and 2c , Supplementary Fig. S2 ), STM 34-2 ( Figs 1a and 2a ), STM 34-7 ( Fig. 1b , Supplementary Fig. S3 ), STM 34-9 ( Fig. 2b , Supplementary Fig. S4 ), IVPP V15564 ( Fig. 2e , Supplementary Fig. S5 ) and IVPP V15036 ( Supplementary Fig. S6 ). 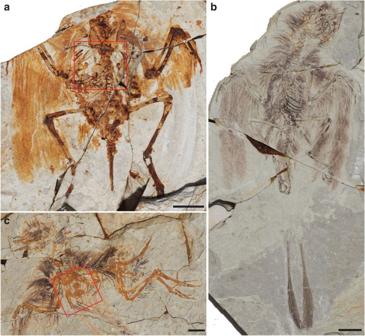Figure 1: New juvenile specimens assigned to Enantiornithes indet. (a) STM 34-2; (b) STM 34-7; (c) STM 34-1. Red box indicates enlarged area inFigure 2. Scale bars, 10 mm. Figure 1: New juvenile specimens assigned to Enantiornithes indet. ( a ) STM 34-2; ( b ) STM 34-7; ( c ) STM 34-1. 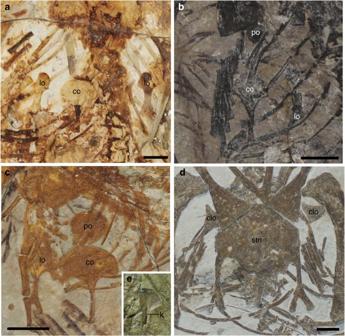Figure 2: Close-up photographs of sternal region of new specimens. (a) STM 34-2; (b) STM 34-9; (c) STM 34-1; (d) DNHM D2522Rapaxavis pani; (e) IVPP V15564A. Anatomical abbreviations: clo, craniolateral ossification; co, caudal ossification; k, keel; lo, lateral ossification; po, proximal ossification; stn, sternum. Scale bars, 5 mm. Red box indicates enlarged area in Figure 2 . Scale bars, 10 mm. Full size image Figure 2: Close-up photographs of sternal region of new specimens. ( a ) STM 34-2; ( b ) STM 34-9; ( c ) STM 34-1; ( d ) DNHM D2522 Rapaxavis pani ; ( e ) IVPP V15564A. Anatomical abbreviations: clo, craniolateral ossification; co, caudal ossification; k, keel; lo, lateral ossification; po, proximal ossification; stn, sternum. Scale bars, 5 mm. Full size image Locality, horizon and age . The specimens all come from different localities of the Early Cretaceous (Aptian) Jiufotang Formation: STM 34-1 is from Liutiaogou, Ningcheng, Chifeng, Inner Mongolia; STM 34-2 is from Dawangzhangzi, Lingyuan, Liaoning; STM 34-7 is from Xisanjia, Ningcheng, Chifeng, Inner Mongolia; and STM 34-9 is from Toudaoyingzi, Jianchang, Liaoning (exception, from the Yixian Formation). IVPP V15564 and V15036 are from the Liutiaogou locality, Ningcheng, Inner Mongolia. Diagnosis . The following skeletal synapomorphies indicate that the specimens are enantiornithine birds: minor metacarpal longer than major metacarpal; Y-shaped furcula; straight scapula; humeral head centrally concave, rising dorsally and ventrally. Differences in proportions of the skeleton and morphologies of the skull and foot suggest that these juveniles belong to different taxa. Despite their diversity, the specimens reveal a consistent pattern of sternal development. Description The preserved sternum of all the new specimens is interpreted as incomplete; we infer that the complete adult sternum was present when the specimen died, but cartilaginous, and only the ossified portions of the element were preserved ( Fig. 3 ). The sternum of IVPP V15564 preserves three ossifications. The largest is caudally located and vertically symmetrical. Proximally, it forms a fan-shaped body with a convex rostral margin; distally it forms a long xiphoid process that always exceeds the rostral body in length. A slight ridge is present on the midline of this ossification, restricted to the caudal half; we infer this to be an early stage in the development of the osseous keel ( Fig. 2e ). This ossification has been previously observed in juvenile enantiornithines (LH 11386, NIGP-130723, GMV 2158, GMV 2159; see Supplementary Table S1 ). IVPP V15564 preserves another ossification on either side of the central element; this bilaterally symmetrical pair forms the lateral trabeculae ( Fig. 3 , Supplementary Fig. S4 ; also visible in GMV-2156/NIGP-130723). These ossifications are typically strap-like with slight expansions at the proximal and distal ends where new growth will occur. In STM 34-2, these ossifications are very wide and robust relative to all other known enantiornithines, and may represent an autapomorphy of the taxon ( Fig. 2a ). 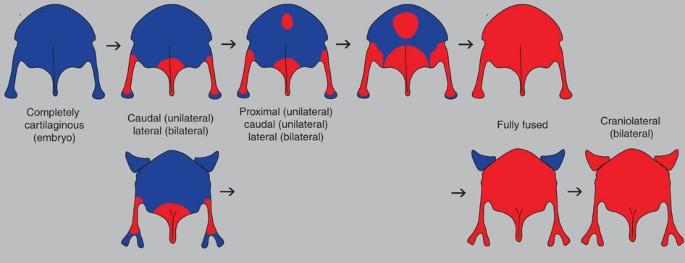Figure 3: Interpretative drawing of the development of the enantiornithine sternum. Red indicates bone and blue indicates cartilage. Figure 3: Interpretative drawing of the development of the enantiornithine sternum. Red indicates bone and blue indicates cartilage. Full size image New specimens STM 34-1, STM 34-7 and STM 34-9 preserve a fourth piece of the sternum that has also not previously been reported. This ossification is a single rounded element located on the midline proximal to the first described (caudal) ossification ( Fig. 2b,c ). In STM 34-7, the proximal ossification is small and oval and located near the rostral margin of the sternum, as inferred by the position of the coracoids (also visible in GMV 2159). STM 34-1 preserves a later ontogenetic stage in which this proximal element is large and more circular; proximally it does not reach the rostral margin of the sternum and distally it remains separate from the caudal ossification ( Fig. 3c ). The lateral ossifications have expanded proximally and medially to contact the caudal midline ossification, although they remain distinctly separate; their distal ends form fork-like expansions. Distally expanded lateral trabeculae are present in most enantiornithines, with varying degrees of complexity; a forked distal expansion was an autapomorphy of Rapaxavis pani [11] ( Fig. 2d ). The caudal ossification has also expanded its body proximolaterally and elongated the xiphoid process. No new ossifications are apparent in this specimen. Although this is the first report of these sternal ossifications, they are preserved in previously described specimens [12] . GMV 2158 and NIGP-130723 preserve the lateral and caudal ossifications. GMV 2159 preserves the caudal, proximal and lateral ossifications. In all these specimens, only the caudal element was identified. Until the discovery of STM 34-1, in which the proximal and lateral ossifications are enlarged, these smaller ossifications went unnoticed. Although it is possible the proximal and caudal unilateral ossifications were originally paired, no specimen possesses a medial suture—present in subadult confuciusornithiforms and jeholornithiforms, whose sterna ossify from a pair of mediolateral plates—suggesting that these are not bilateral ossifications. The holotype specimens of Rapaxavis pani (DNHM D2522) and Concornis lacustris (LH 2814), the former a subadult specimen, both preserve an additional pair of ossifications ( Fig. 2d ). In these specimens, the sternum is only represented by three parts; the four previously identified ossifications are inferred to be completely fused into a single element, preserved together with a new bilaterally symmetrical pair of ossifications. Previously termed the paracoracoidal ossifications [11] , these bones are clearly associated with the sternum and resemble in form and topology the craniolateral processes of the sternum in modern birds [13] . This pair of ossifications has also been identified in an undescribed specimen, STM 11-188 ( Supplementary Fig. S7 ). In no specimen are these ossifications fused to the sternum, and it is possible they remained associated only through ligamental or cartilaginous connections. Their presence in a limited number of specimens suggests either they independently arose in one or more enantiornithine lineages, convergent with ornithurines, or that they appear very late in ontogeny and are either not preserved in subadults or are lost due to the absence of complete fusion with the body of the sternum. Given that the very small early sternal ossifications are preserved in young juveniles, loss due to preservation is not considered probable. Understanding the development of a complex skeletal element can help us to better understand its origin, homology and function [9] , [10] . The sternum of Cretaceous ornithurines, the clade that includes living birds, is essentially modern in appearance, preserving all major structural features that are present in neornithines (for example, rostrally projecting, ventrally deep keel, deep coracoidal sulci, rostral spine, craniolateral processes, caudal fenestrae). How this complex element evolved from the two simple plates observed in most non-avian dinosaurs is unclear ( Fig. 4 ). Direct comparison with Cretaceous ornithuromorphs is hindered by the absence of known juvenile specimens preserving early ontogenetic stages. The evolution of derived features (for example, caudolateral process) and secondary loss of plesiomorphic neornithine features (for example, keel) over 65 million years makes it difficult to construct generalizations regarding the development of the sternum in living birds [13] . We also recognize that the developmental pathways that lead to a superficial morphotype may have changed through time and in clade-specific ways. Furthermore, a majority of recent research on living birds focuses on embryological development [4] , [5] , [14] , [15] , [16] , [17] , [18] , which is poorly known for extinct taxa. However, a review of literature dating back over a century creates the basis for comparison with enantiornithines [5] , [6] , [8] , [13] , [14] , [16] , [19] . 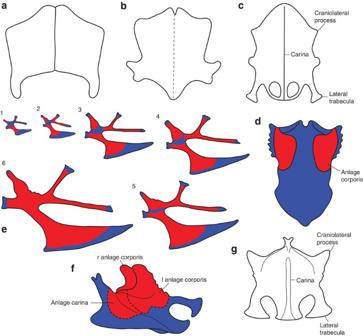Figure 4: Developing and adult sternal morphology in Maniraptora. (a) Reconstruction of the sternum ofLinheraptor exquisitus(Theropoda; Dromaeosauridae) showing two sternal plates; (b) reconstruction of the sternum ofConfuciusornis sanctus(Aves: Pygostylia)—the dashed line indicates a suture present in some specimens; (c) reconstruction of the sternum ofYixianornis grabaui(Aves: Ornithuromorpha); (d) development of the sternum ofCasuarius bennettii, showing two pairs of ossification centres (modified from Parker8); (e) the sternum ofMerula vulgaris(Neornithes: Passeriformes; modified from Parker8); (f) the development of the sternum ofMerula, showing the three ossification centres (modified from Parker8); G1–6, six stages in the development of the sternum ofChryodophus amerherstiae(Neornithes: Galliformes) showing the craniolateral and caudolateral processes forming from separate ossification centres (modified from Wen and Yang16). Red indicates bone and blue indicates cartilage. Figure 4: Developing and adult sternal morphology in Maniraptora. ( a ) Reconstruction of the sternum of Linheraptor exquisitus (Theropoda; Dromaeosauridae) showing two sternal plates; ( b ) reconstruction of the sternum of Confuciusornis sanctus (Aves: Pygostylia)—the dashed line indicates a suture present in some specimens; ( c ) reconstruction of the sternum of Yixianornis grabaui (Aves: Ornithuromorpha); ( d ) development of the sternum of Casuarius bennettii , showing two pairs of ossification centres (modified from Parker [8] ); ( e ) the sternum of Merula vulgaris (Neornithes: Passeriformes; modified from Parker [8] ); ( f ) the development of the sternum of Merula , showing the three ossification centres (modified from Parker [8] ); G1–6, six stages in the development of the sternum of Chryodophus amerherstiae (Neornithes: Galliformes) showing the craniolateral and caudolateral processes forming from separate ossification centres (modified from Wen and Yang [16] ). Red indicates bone and blue indicates cartilage. Full size image Enantiornithes is sister group to Ornithuromorpha, which together form the clade Ornithothoraces. Although ornithothoracine sterna are superficially similar and far more derived than other groups of Mesozoic birds (for example, Confuciusornithiformes, Jeholornithiformes), enantiornithines retain some basal morphologies (for example, poorly developed keel). Basal ornithuromorphs and enantiornithines show similar sternal morphologies, which suggests the fully modern sternum evolved only among more derived members of Ornithuromorpha, the Ornithurae ( Fig. 4c,e ). Unfortunately, no early juvenile ornithurines are recognized; however, given the derived appearance of the sternum we infer that development may have proceeded similarly to that of living birds. This is supported by the ossification of the sternum from a single pair of plates in most paleognaths [8] , [14] , indicating the plesiomorphic dinosaurian condition was retained in the lineage leading to modern birds ( Fig. 4d ). Enantiornithines are already known to have a developmental strategy different from most living birds in which they grew slowly for many years [20] , [21] , [22] , and spent extended periods of time as subadults, as evidenced from the large number of juvenile and subadult specimens uncovered (see Methods). These specimens reveal early ontogenetic stages that allow us to understand the skeletal development of the clade. What has become apparent from this study is that, despite its superficially similar appearance, the enantiornithine sternum formed very differently from that of non-avian dinosaurs and living birds. As in living birds, the basal bird sternum was incompletely ossified in juveniles [6] , [8] . The sternum of enantiornithines developed from four to six ossifications ( Fig. 3 ). As in the morphological description, the sternal ossifications of enantiornithines will be referred to by their positions: proximal, caudal, lateral (paired) and craniolateral (paired, variably present). Although we will attempt to correlate these with ossification centres observed in living birds, the apparent lack of homology causes us to refrain from naming these ossifications according to previous literature [8] , [13] . Given the diversity in the number of ossification centres in living taxa (two to seven) [8] , it would not be unexpected that there is similar diversity within Enantiornithes. This suggests the presence of craniolateral ossifications in only a few enantiornithines may be related to lineage-specific specialization of the sternum. Given the area left unossified in STM 34-1, the latest recognized stage before the sternal body ossifies into a single element, it is possible another pair of ossifications may have existed, forming the costal region ( Fig. 2c ). However, given that they have not yet appeared in STM 34-1 despite the expansion of all other ossifications that contribute to the sternal body, we suggest that it is not likely. Ossification proceeds from the caudal half proximally, which is opposite to the direction of sternal development in living birds [6] , [8] , [13] ( Fig. 4d,f,g ). The main body of the sternum in enantiornithines is formed by two ossifications, as in birds and non-avian dinosaurs, but instead of a bilaterally symmetrical pair, they are two proximo-distally arranged vertically symmetrical ossifications of very different morphology. Basal maniraptoran taxa and juvenile specimens, as well as several other groups of dinosaurs (for example, ceratopsians, ornithopods, sauropods) [23] , possess a pair of medially unfused sternal plates ( Caudipteryx, Bambiraptor, Linheraptor ; Fig. 4a ); in more derived maniraptorans (and adult specimens) these plates fuse and form a unified sternum ( Microraptor ). Although Jeholornis and Confuciusornis both possess a single quadrangular sternal element, some specimens preserve clefts on the rostral and caudal midline connected by a visible medial suture ( Confuciusornis STM 13-242, STM 13-203; Jeholornis STM 2-39, STM 2-16), indicating the sternum developed from a pair of plates, as in closely related maniraptoran dinosaurs ( Fig. 4b ). Living birds also possess a bilateral pair of ossifications primarily responsible for the body of the sternum (anlage corporis of Livezy and Zusi [13] and pleurosteon of Parker [8] ). In the flightless ratites with the exception of Rhea , the sternum forms entirely from a single pair of ossifications [8] , apparently the same as in non-avian dinosaurs. This pair appears during embryological development, widely separated mediolaterally, and do not fully expand to meet and fuse into a single element until late in ontogeny [8] , [14] . The absence of additional sternal ossifications among ratites is inferred to be secondary, lost when the group evolved to be flightless [1] , [8] . The enantiornithine condition, in which the majority of the sternum is formed by two unilateral ossifications, is very different from both the dinosaurian and neornithine pattern of development: formed primarily from bilateral pairs of ossifications. The presence of unilateral sternal ossifications within Aves is not unprecedented; the development of the carina is in some cases believed to derive from a single ossification (lophosteon, Parker) and a single distal ossification centre that forms the caudal margin of the sternum has been reported in some taxa (urosteon, Parker) [8] . The development of the lateral trabeculae from an independent pair of ossifications is consistent with some groups of living birds (for example, Galliformes, Corvus ). Within Neornithes, this process is variably present in different groups and similarly positioned processes of uncertain homology exist (for example, caudolateral process; Fig. 4c,e–g ). In most cases, this process appears to be formed by an extension of the corporis ossification [8] , [13] . Galliformes possess a pair of large forked caudal processes sometimes considered the caudal trabeculae ( Fig. 4g ); similar to enantiornithines, this part of the sternum forms from a separate pair of ossifications (mesosteon of Parker; anlage caudo-lateralis of Livezy and Zusi) [8] , [13] . Early Cretaceous ornithuromorphs ( Fig. 4c ) possess lateral trabeculae of comparable morphology to living taxa where the process ossifies from the corporis (for example, Merula – Fig. 4e , Cairina ) [5] , [8] . The morphology of the 'caudal trabeculae' in Cretaceous ornithothoracines, although similar in that they extend to approximately the caudal margin of the sternum and an intermediate pair is additionally present, also differ greatly; the ornithuromorph trabeculae extend to the same level and in some cases enclose fenestrae, whereas in enantiornithines the lateral trabeculae demarcate deep caudal embayments with the xiphoid process and the intermediate trabeculae are very short. These differences in morphology as well as ossification suggest the observed similarities represent parallelisms within the ornithothoracines. This is also documented in another basal clade of birds, the Jeholornithiformes [24] , [25] , and at least one dromaeosaurid also preserves an elongate pair of 'caudal trabeculae' ( Linheraptor — Fig. 4a ). In juvenile enantiornithines, the keel appears to have developed as an extension of the caudal ossification (IVPP V15564; STM 34-1; Fig. 2e ). The adult enantiornithine keel is low and caudally restricted in all known specimens, with the exception of the derived Late Cretaceous Neuquenornis volans , where it is deep and rostrally projecting as in ornithurines and modern flighted birds [26] . The absence of a deep keel in Early Cretaceous enantiornithines is considered real, as opposed to preservational, given the wide distribution of a deep keel preserved in sympatric Jehol ornithuromorphs (for example, Yixianornis , Yanornis ). All living flighted birds preserve an ossification for the carina that forms proximally and progresses distally (lophosteon of Parker; anlage carina of Livezy and Zusi) [8] , [13] , [16] . Although preservation and identification of a ventrally located ossification of the carina would be difficult, its absence in all known juvenile specimens together with the morphology of the Early Cretaceous enantiornithine sternum suggests this ossification was not present in this group. However, the morphology in Neuquenornis suggests it may have evolved later within the clade, in parallel with ornithurines. Alternatively, in Neuquenornis the keel may have developed from an extension of an existing ossification. Interestingly, in some living birds the carina ossification has expanded to form not only the keel but also a large extent of the sternal body [8] . The craniolateral ossifications present in Concornis and Rapaxavis resemble the craniolateral processes of the sternum in ornithurine birds in morphology and topology. In Rapaxavis ( Fig. 2d ), where preservation is clearest, the ossifications do not contribute to any other morphologies of the sternum, only forming a rostrodorsal proximally tapering projection that we suggest would have served a similar function as the process in living birds. In most neornithine taxa, this process is relatively small and forms from an extension of the sternal body [8] . The enantiornithine condition resembles Rhea ; besides the main pair of ossifications that form the sternum in other ratites, Rhea possesses an additional pair that form distinct craniolateral processes (pro-osteon, Parker) [8] , [14] . However, in this taxon the ossifications also form the costal margin and are fused to the sternal body [8] . A similar morphology is present in the Galliformes ( Fig. 4g ). Thus, it appears that distinct, separately ossifying craniolateral processes evolved several times within Aves, in Enantiornithes and potentially more than once within Neornithes, in Palaeognathae and Neognathae. Craniolateral extension of the sternum may have been important not only to the flight stroke as similar small processes are observed on the sternum of at least one oviraptorosaur ( Citipati ) [27] . Their developmental origin in this group remains unclear; so far there is only evidence for a single pair of sternal ossifications present in non-avian dinosaurs ( Fig. 5 ). 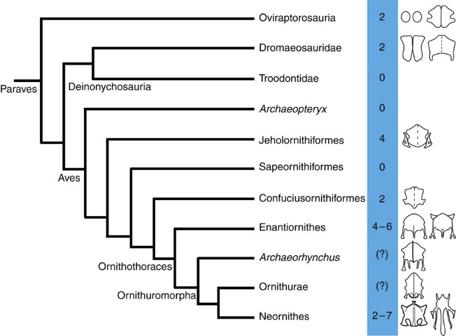Figure 5: Cladogram of sternal morphologies and ossifications. Sternal morphologies and the inferred number of ossifications presented across a simplified cladogram of paravian relationships. Example sterna: Oviraptorosauria,CaudipteryxandCitipati; Dromaeosauridae,BambiraptorandMicroraptor; Jeholornithiformes,Jeholornis prima; Confuciusornithiformes,Confuciusornis sanctus; Enantiornithes,LongipteryxandRapaxavis; Ornithurae,Yixianornis; Neornithes,MerulaandGallus. Dashed lines indicate regions where two ossifications become fused. Figure 5: Cladogram of sternal morphologies and ossifications. Sternal morphologies and the inferred number of ossifications presented across a simplified cladogram of paravian relationships. Example sterna: Oviraptorosauria, Caudipteryx and Citipati ; Dromaeosauridae, Bambiraptor and Microraptor ; Jeholornithiformes, Jeholornis prima ; Confuciusornithiformes, Confuciusornis sanctus ; Enantiornithes, Longipteryx and Rapaxavis ; Ornithurae, Yixianornis ; Neornithes, Merula and Gallus . Dashed lines indicate regions where two ossifications become fused. Full size image Several features considered homologous between enantiornithines and more derived birds are now demonstrated to have very different developmental origins. The occurrence of similar features in isolated species of distantly related groups (for example, caudal trabeculae in dromaeosaurids and craniolateral processes in oviraptorosaurs) highlights the plasticity of the sternum and suggests the presence of similar physical forces acting on different groups to produce parallel morphologies ( Fig. 5 ). The distribution of dinosaur sterna suggests that their presence is plesiomorphic in Aves; the ornithothoracine common ancestor probably possessed paired sternal plates, medially fused in the adult. However, given the absence of a sternum in some Mesozoic birds ( Archaeopteryx , Sapeornis ), it is possible that the ornithothoracine common ancestor did not have an ossified sternum. The condition in Enantiornithes is inferred to be an autapomorphy of the clade; developmental and morphological differences between the two clades suggest that shared features of the ornithothoracine sternum were not present in their common ancestor. The assumption of primary homology for many features despite morphological differences, such as those of the sternum and potentially the coracoid and pygostyle, is largely the basis for the sister relationship between Enantiornithes and Ornithuromorpha. However, the developmental differences highlighted by this study suggest that morphological similarities may represent parallelism and the close relationship between these two clades may need to be re-examined. Material New material used for this study includes six previously undescribed juvenile specimens (fledglings) assigned to Enantiornithes indet. : STM 34-1 ( Figs 1c and 2c , Supplementary Fig. S1 ), STM 34-2 ( Figs 1a and 2a ), STM 34-7 ( Fig. 1b , Supplementary Fig. S3 ), and STM 34-9 ( Fig. 2b , Supplementary Fig. S2 ) housed at the Tianyu Natural History Museum, Shandong, China and IVPP V15564 ( Fig. 2e , Supplementary Fig. S4 ) and IVPP V15036 ( Supplementary Fig. S5 ) housed at the Institute of Vertebrate Paleontology and Paleoanthropology, Beijing, China. The specimens are identified as juveniles based on their size (much smaller than adult enantiornithines), incomplete ossification of skeletal elements (sternum, pygostyle), and proportions (for example, large orbit). Several previously described specimens are also incorporated in this study: GMV 2158—juvenile enantiornithine indet. [12] housed at the Geological Museum of Beijing, China; GMV 2159—juvenile enantiornithine indet. [12] GMV 2156/NIGP-130723—juvenile enantiornithine, former holotype of Liaoxiornis delicatus and Lingyuanornis parvus , respectively [12] , [28] , [29] (the latter is housed at the Nanjing Institute of Geology and Paleontology, Nanjing, China); IVPP V12552—subadult Longipteryx chaoyangensis [30] ; DNHM D2522—holotype of Rapaxavis pani , subadult [31] , [32] ( Fig. 2d ) housed at the Dalian Natural History Museum, Dalian, China; and LH 2814 - holotype of Concornis lacustris , housed at the Museo de las Ciencias de Castilla-La Mancha, Cuenca, Spain [33] . Enantiornithine developmental strategy The precocial–altricial spectrum is the range of developmental strategies occupied by living birds, from largely independent to fully dependent on their parents; developmental strategy affects the degree of ossification and feathering in hatchlings, although other characteristics such as egg size and incubation time do not show strong correlation [33] . The enantiornithine developmental strategy is described as precocial or super-precocial [34] . Remiges (flight feathers of the wings) are preserved in an embryo and numerous young juveniles [34] . In living birds, only the 'super-precocial' megapodes are born fledged and capable of flight [33] , thus the presence of fully developed remiges on young enantiornithines may suggest independence from adults. One specimen (STM 34-7) even preserves paired caudal rectrices suggesting the presence of adult or near adult plumage. Early enantiornithine juveniles and embryos also show a high degree of ossification, indicative of precociality in living birds [35] . Although limited histological work has been conducted, what is apparent for the clade is that they grew rapidly during embryology and slowly after hatching. The large number of early juvenile enantiornithine specimens that have been collected (an ontogenetic period that is not recorded for any other clade of Mesozoic birds) leads to the interpretation that the postnatal period was prolonged in these birds [21] , [22] . After reaching adult morphology, enantiornithines continued to grow for an extended (but unknown) period of time, as evidenced from the preservation of several lines of arrested growth in adult specimens [36] . In living birds the postnatal period lasts anywhere from 2 months to several years, although typically maturation is complete within a year [33] , and only the Kiwi has lines of arrested growth [37] , [38] . Although most definitely precocial, enantiornithines probably do not fall within the neornithine altricial-precocial spectrum (differences in growth strategy, restrictions in egg size because of distally contacting pubes). Several aspects of precociality (degree of parental care) remain unknown for enantiornithines. However, for observable features (degree of feathering and ossification at hatching), enantiornithines are more comparable to living precocial birds (feathered and highly ossified) than to those that are altricial (naked, relatively less ossified). Subadult enantiornithines close to complete in their skeletal development are nearly adult in size (10% smaller) but the carpometacarpus and tarsometatarsus remain unfused ( Longipteryx IVPP V12352, Shenqiornis DNHM D2950/1, Rapaxavis DNHM D2522) [22] . In the absence of histology, we can only estimate from the incomplete ossification of several important features that the specimens described here are relatively early in their postnatal development. Distribution of sterna in archosauria Sterna are present in a wide diversity of vertebrates; in reptiles the sternum consists embryologically of a pair of cartilaginous plates located caudal to the coracoids, articulating with the cranial thoracic ribs [39] . Within Archosauria, sternal plates are present in Pterosauria and Dinosauria ( Supplementary Fig. S1 ). Pterosaurs, being also adapted for flight, have well-developed fused sterna with a large rostroventrally projecting carina [40] . Within Dinosauria paired sternal plates are present in the ornithomimosaur Pelicanomimus , pro-sauropods, sauropodomorphs, Stegasaurus , ankylosaurs (partially fused in some taxa), basal ornithopods, hadrosaurs, pachycephalosaurs, basal ceratopsians, ceratopsids, the basal ceratosaur Limusaurus (fused) and maniraptorans ( Supplementary Fig. S1 ) [23] , [41] . Sternal plates are present in a number of maniraptoran clades [42] . Alvarezsaurs have well-developed sterna related to their unique specialization of the forelimb; the sternum is fully fused and possesses a large ventral keel [43] . No therizinosauroid has yet to preserve sternal elements although their presence is inferred [44] . Within Oviraptorosauria, basal taxa have simple oval plates that may or may not have contacted medially ( Caudipteryx ); more derived taxa have medially articulating sternal plates that form a quadrangular sternum ( Citipati , Oviraptor ) [27] , [45] . Some specimens have craniolateral processes and lateral processes ( Citipati , Oviraptor ) and one taxon may have had a fully fused sternum ( Ingenia ) [46] . Paraves is the maniraptoran clade that includes birds and their closest dinosaurian relatives: Dromaeosauridae, Troodontidae and Scansoriopterygidae. Dromaeosauridae encompasses a number of sternal morphologies although they are typically simple, paired, medially articulating, proximo-distally elongate elements [47] . In some cases they are medially fused, a feature that is affected by ontogeny ( Microraptor ; personal observation). Small craniolateral processes ( Microraptor , TMP 92.36.333), costal facets (TMP 92.36.333) or elongate caudal 'trabeculae' ( Linheraptor ) are all known to occur in the clade, although none of these features co-occur in a single specimen (although all these features are present in ornithuromorphs and some enantiornithines) [48] , [49] . Members of Troodontidae appear to not have ossified sternal plates [50] . Within Scansoriopterygidae, sternal elements are reported but poorly preserved only in Epidexipteryx [51] . How to cite this article: Zheng, X. et al . Insight into the early evolution of the avian sternum from juvenile enantiornithines. Nat. Commun. 3:1116 doi: 10.1038/ncomms2104 (2012).